Antibiotic-induced shifts in the mouse gut microbiome and metabolome increase susceptibility toClostridium difficileinfection Antibiotics can have significant and long-lasting effects on the gastrointestinal tract microbiota, reducing colonization resistance against pathogens including Clostridium difficile . Here we show that antibiotic treatment induces substantial changes in the gut microbial community and in the metabolome of mice susceptible to C. difficile infection. Levels of secondary bile acids, glucose, free fatty acids and dipeptides decrease, whereas those of primary bile acids and sugar alcohols increase, reflecting the modified metabolic activity of the altered gut microbiome. In vitro and ex vivo analyses demonstrate that C. difficile can exploit specific metabolites that become more abundant in the mouse gut after antibiotics, including the primary bile acid taurocholate for germination, and carbon sources such as mannitol, fructose, sorbitol, raffinose and stachyose for growth. Our results indicate that antibiotic-mediated alteration of the gut microbiome converts the global metabolic profile to one that favours C. difficile germination and growth. C lostridium difficile is an anaerobic, spore-forming, Gram-positive bacillus first isolated in 1935 (ref. 1 ). Within the past decade, new focus has been put on C. difficile owing to an increase in morbidity, mortality and health-care costs associated with infection by this pathogen [2] , [3] . Hospitalization, age greater than 65 years and antibiotic treatment are the primary risk factors for C. difficile infection (CDI) [4] , [5] . Antibiotics are a key risk factor in the pathogenesis of CDI, as these drugs have significant and long-lasting effects on the intestinal microbiota [6] , [7] , which are associated with reduced colonization resistance against pathogens, including C. difficile [8] , [9] . Colonization resistance is the ability of the indigenous gut microbiota to prevent colonization by pathogens [10] , [11] . The mechanisms by which antibiotics lead to a loss of colonization resistance are unknown and probably reflect changes in the ecologic, metabolic and immunologic functions of the intestinal microbiome/host ecosystem. By altering the structure of the gut microbiome, antibiotics alter the function of this community. This change in function is reflected in the intestinal metabolome, which includes both host- and microbial-derived metabolites. The intestinal microbiota plays a major role in the fermentation of complex carbohydrates and amino acids into short-chain fatty acids (SCFAs) that are important for colonic health [12] , [13] , [14] . The intestinal microbiome also plays a role in lipid metabolism, amino-acid metabolism and protein digestion [15] , [16] , [17] , [18] . Alteration of the metabolic activity of the microbiome via antibiotics is posited to facilitate growth of enteric pathogens [19] . We hypothesize that changes in the structure and function of the gut microbial community after antibiotic treatment creates a metabolic environment that favours C. difficile germination and growth. The spore form of C. difficile is dormant until it encounters germinants, including bile acids, which initiate outgrowth of vegetative cells [20] . These vegetative bacteria produce the main virulence factors of C. difficile , the toxins TcdA and TcdB, in late stationary phase, resulting in epithelial damage [21] . It has been observed that the levels of glucose and other nutrients affect expression of C. difficile toxin genes [21] . To study the complex interaction between this pathogen, the microbiome and the metabolome, we used a combination of 16S ribosomal RNA gene sequencing and mass spectrometry to define the structural and functional changes in the gastrointestinal tract environment that accompany the loss and restoration of colonization resistance in a murine model of CDI [9] , [22] . Here we show that susceptibility to CDI following antibiotic administration is associated with distinct shifts in the gastrointestinal microbiome and metabolome. By following the dynamics of the gut ecosystem after antibiotic treatment, we identify multiple states of the gastrointestinal ecosystem that are resistant to CDI. These states have distinct microbial community structures but similar metabolic function. The metabolic environment of the murine gastrointestinal tract after antibiotic treatment is enriched in primary bile acids and carbohydrates that support germination and growth of C. difficile in vitro and ex vivo . This report illustrates how the structure of the gut microbiome can shape community function and ultimately influence disease outcome. Antibiotics alter the structure of the gut microbiome We previously demonstrated that treatment of mice with the broad-spectrum antibiotic cefoperazone reproducibly shifts the gut microbiome into distinct structural states in terms of microbiota composition [6] . Furthermore, these states differ functionally based on colonization resistance to C. difficile [9] . At the baseline state (without antibiotic treatment), mice exhibit complete colonization resistance against C. difficile . Two days after completing a 10-day course of cefoperazone, the gut ecosystem of these mice was in a state fully susceptible to CDI. However, once mice were given 6 weeks to recover from cefoperazone treatment, the gut returned to a state of complete colonization resistance against C. difficile . To further define the intestinal environment that characterized susceptibility and resistance to C. difficile , we treated additional groups of wild-type (WT) C57BL/6 mice with cefoperazone. Following all treatments, animals in each group were split into two sets. Tissue and intestinal contents from one set was harvested for microbiome and metabolome characterizations, while animals in the other set were challenged with C. difficile spores to evaluate susceptibility to CDI ( Supplementary Fig. 1 ). Two days after cefoperazone treatment, the intestinal environment was in a state fully susceptible to C. difficile colonization (designated S1 in Fig. 1 ). This state was characterized by significant changes in the composition and diversity of the gut microbiome ( Supplementary Fig. 2 ). Interestingly, changes in the total bacterial load were not significant when compared with non-antibiotic-treated mice (R1) suggesting that colonization resistance was dependent on the specific structure of the community and not simply overall community size ( Supplementary Fig. 2a ). Six weeks after cefoperazone treatment, the intestinal environment returned to a state of full colonization resistance ( Fig. 1 , R3); however, the community structure of the microbiome associated with this state differed from that encountered in non-antibiotic-treated mice ( Fig. 1 , R1–R2; Supplementary Figs 3 and 4 ). These non-antibiotic-treated baseline states were indistinguishable by microbiome structure indicating stability over a 6-week period ( Supplementary Fig. 4 ). 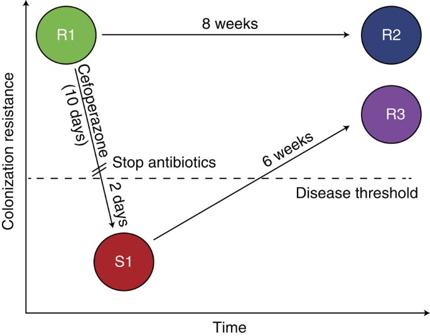Figure 1: Susceptible and resistant states of CDI. Each circle represents the state of the intestinal environment for each of the four treatment groups. C57BL/6 wild-type mice (represented at baseline by state R1) were treated with cefoperazone for 10 days. The structural and functional status of the gut was determined 2 days (S1) or 6 weeks (R3) after discontinuation of the antibiotic. An additional group of mice (R2) was held without any antibiotic treatment to serve as age-matched controls to the R3 animals. Each treatment group was challenged withC. difficilespores to assess whether they were resistant or susceptible to colonization and disease. There were three states that were fully resistant to colonization and disease (R1, R2 and R3) and one susceptible state (S1). Figure 1: Susceptible and resistant states of CDI. Each circle represents the state of the intestinal environment for each of the four treatment groups. C57BL/6 wild-type mice (represented at baseline by state R1) were treated with cefoperazone for 10 days. The structural and functional status of the gut was determined 2 days (S1) or 6 weeks (R3) after discontinuation of the antibiotic. An additional group of mice (R2) was held without any antibiotic treatment to serve as age-matched controls to the R3 animals. Each treatment group was challenged with C. difficile spores to assess whether they were resistant or susceptible to colonization and disease. There were three states that were fully resistant to colonization and disease (R1, R2 and R3) and one susceptible state (S1). Full size image Antibiotics alter the function of the gut metabolome We explored the gastrointestinal metabolome associated with each of the functional states of the intestinal ecosystem using an untargeted approach. Caecal contents from the unchallenged sets of animals ( Supplementary Fig. 1a ) were analysed by multiple mass spectrometry platforms, identifying a total of 480 metabolites from a library of 2,400 known biochemical compounds [23] . The metabolome of the state susceptible to CDI ( Fig. 1 , S1) was characterized by significant changes to metabolites belonging to the following Kyoto Encyclopedia of Genes and Genomes metabolic pathways: amino acids, carbohydrates, lipids, peptides and xenobiotics when compared with the initial states resistant to CDI ( Fig. 1 R1–R2; Fig. 2a ; Supplementary Figs 5 and 6a ; Supplementary Data 1 ). Similarly, the gut metabolome associated with the state of C. difficile susceptibility was drastically different from the resistant state encountered 6 weeks after cefoperazone treatment ( Fig. 1 , R3; Supplementary Figs 5 and 6b,c and Supplementary Data 2 ). Both non-antibiotic-treated baseline states ( Fig. 1 , R1–R2) had almost identical metabolic profiles, demonstrating stability of the gut metabolome over a 6-week period that reflected the stability of community structure ( Supplementary Fig. 6d ). 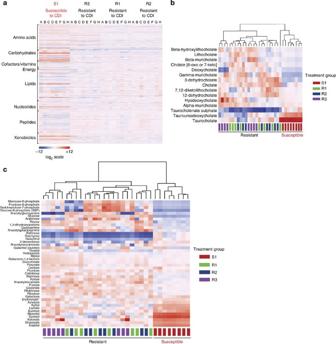Figure 2: Untargeted metabolomics of the gut metabolome. (a) A heatmap of the metabolites grouped by Kyoto Encyclopedia of Genes and Genomes pathway found in the gut metabolome of CDI-susceptible and -resistant mice from all four treatment groups (n=8, A–H). Mice susceptible to CDI (S1) showed significant changes in their intestinal metabolome compared with the three groups of mice with intestinal environments that were resistant toC. difficilecolonization (R1–R3). (b) A heatmap of the relative amounts of bile acids in the gut metabolome of CDI-susceptible and -resistant mice from all four treatment groups. The heatmap scale ranges from −6 to +8 on a log2scale. (c) A heatmap of carbohydrates in the gut metabolome of CDI-susceptible and -resistant mice from all four treatment groups. The heatmap scale ranges from −5 to +10 on a log2scale. Figure 2: Untargeted metabolomics of the gut metabolome. ( a ) A heatmap of the metabolites grouped by Kyoto Encyclopedia of Genes and Genomes pathway found in the gut metabolome of CDI-susceptible and -resistant mice from all four treatment groups ( n =8, A–H). Mice susceptible to CDI (S1) showed significant changes in their intestinal metabolome compared with the three groups of mice with intestinal environments that were resistant to C. difficile colonization (R1–R3). ( b ) A heatmap of the relative amounts of bile acids in the gut metabolome of CDI-susceptible and -resistant mice from all four treatment groups. The heatmap scale ranges from −6 to +8 on a log 2 scale. ( c ) A heatmap of carbohydrates in the gut metabolome of CDI-susceptible and -resistant mice from all four treatment groups. The heatmap scale ranges from −5 to +10 on a log 2 scale. Full size image The gut metabolome of the susceptible S1 state was associated with relative increases in primary bile acids, including taurocholate and other tauro-conjugated bile acids, while levels of the secondary bile acid deoxycholate decreased ( Fig. 2b ). With regard to carbohydrates, sugar alcohols increased in the gut metabolome of the state susceptible to CDI while those in the glycolytic pathway decreased ( Fig. 2c ). The most significant increase in carbohydrates was seen in the sugar alcohols mannitol (553-fold) and sorbitol (1,053-fold). Other polyols that increased in the gut after antibiotics were arabitol, xylitol and ribitol. The increase in available carbohydrates in state S1 coincided with a significant decrease in free short-, medium- and long-chain fatty acids ( Supplementary Data 1 ). The SCFA valerate decreased 66-fold after antibiotic treatment. The decrease in SCFAs and increase in available carbohydrates suggests a decrease in carbohydrate fermentation by members of the gut microbiota. Six weeks after discontinuation of antibiotics, carbohydrate levels returned to baseline along with most fatty acids. The state of susceptibility to CDI was characterized by increases in amino acids including ones required for C. difficile germination and growth: glycine, proline, cysteine, isoleucine, valine, leucine and tryptophan ( Supplementary Data 1 ) [24] . This state also demonstrated a 28-fold decrease in the branch-chained fatty-acid isovalerate, which is a marker for protein digestion in the gut [25] . Proteases and peptidases from the indigenous gut microbiota and host play an important role in degradation of proteins into smaller peptides and amino acids [18] . Antibiotic treatment resulted in a significant decrease in luminal dipeptides, although most levels returned to baseline 6 weeks after discontinuing cefoperazone treatment, suggesting the return of specific members of the gut microbiome could be important for protein digestion. Although the relative levels of dipeptides were returning to baseline after 6 weeks, amino acids did not ( Supplementary Data 2 ). Confirmation of gut metabolome shifts using a targeted approach To more precisely define the changes in the gut metabolome identified using the untargeted metabolomics approach, we used a targeted metabolomics approach to measure the concentrations of bile acids, sugar alcohols and SCFAs. Untargeted metabolomics analysis indicated that loss of colonization resistance (S1) was associated with relative increases in primary bile acids and a corresponding decrease in secondary bile acids. Direct measurement of bile acids confirmed these results ( Fig. 3a ). Before antibiotics, the secondary bile acids deoxycholate and cholate were detected at 6.45 and 2.15 μg per 100 mg of caecal content, respectively. Following antibiotic treatment, the secondary bile acid deoxycholate was below the limit of detection while the primary bile acids taurocholate and cholate were detected at 8.02 μg and 0.22 μg per 100 mg of caecal content, respectively. 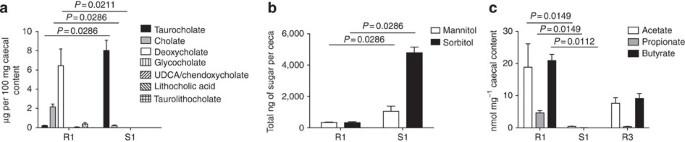Figure 3: Targeted metabolomics of gut metabolome. (a) Bile acids were analysed by LC-MS from the caecal content of non-antibiotic-treated (R1) and cefoperazone-treated mice (S1) (n=4 for each group). Significant changes in the concentrations of taurocholate, cholate and deoxycholate resulted from antibiotic treatment (the Mann–Whitney non-parametrict-test). Error bars represent the mean±s.e.m. (b) Concentrations of sugar alcohols (mannitol and sorbitol) measured by LC-MS from caecal content of untreated (R1) and cefoperazone-treated mice (S1) (n=4 for each group). Antibiotic treatment significantly changes the levels of these sugar alcohols (the Mann–Whitney non-parametrict-test). Error bars represent the mean±s.e.m. (c) SCFA levels (acetate, propionate and butyrate) were analysed by gas chromatography/mass spectroscopy from caecal content of non-antibiotic-treated (R1,n=3), 2 days (S1,n=4) and 6 weeks after cefoperazone-treated mice (R3,n=3). Changes in SCFAs were significant between groups R1 and S1 (the non-parametric Kruskal–Wallis one-way analysis of variance test followed by Bonferroni–Dunn multiple comparison test). Error bars represent the mean±s.e.m. Figure 3: Targeted metabolomics of gut metabolome. ( a ) Bile acids were analysed by LC-MS from the caecal content of non-antibiotic-treated (R1) and cefoperazone-treated mice (S1) ( n =4 for each group). Significant changes in the concentrations of taurocholate, cholate and deoxycholate resulted from antibiotic treatment (the Mann–Whitney non-parametric t -test). Error bars represent the mean±s.e.m. ( b ) Concentrations of sugar alcohols (mannitol and sorbitol) measured by LC-MS from caecal content of untreated (R1) and cefoperazone-treated mice (S1) ( n =4 for each group). Antibiotic treatment significantly changes the levels of these sugar alcohols (the Mann–Whitney non-parametric t -test). Error bars represent the mean±s.e.m. ( c ) SCFA levels (acetate, propionate and butyrate) were analysed by gas chromatography/mass spectroscopy from caecal content of non-antibiotic-treated (R1, n =3), 2 days (S1, n =4) and 6 weeks after cefoperazone-treated mice (R3, n =3). Changes in SCFAs were significant between groups R1 and S1 (the non-parametric Kruskal–Wallis one-way analysis of variance test followed by Bonferroni–Dunn multiple comparison test). Error bars represent the mean±s.e.m. Full size image Direct measurement of mannitol and sorbitol by liquid chromatography/mass spectroscopy (LC-MS) confirmed significant increases in the levels of these sugar alcohols after antibiotic treatment ( Fig. 3b ). In contrast to the increases in sugar alcohols, measurement of the SCFAs acetate, propionate and butyrate by gas chromatography/mass spectroscopy confirmed significant decreases in the levels of these organic acids after antibiotic treatment ( Fig. 3c ). Six weeks after discontinuing antibiotics, the level of SCFAs had increased. These changes in levels of carbohydrates and fatty acids after antibiotic treatment probably reflect changes in fermentative activity of the gut microbiota. A metabolic environment that favours germination and growth Antibiotic treatment resulted in a shift in the bile salt composition, from secondary bile acids such as deoxycholate to primary bile acids including taurocholate ( Fig. 3a ). Each of these bile salts were tested for the ability to promote germination of C. difficile VPI 10463 spores ( Fig. 4a ). When tested at either the high concentration commonly used for germination assays [20] or the lower concentration observed in our targeted metabolomics studies, significantly higher levels of germination were evident in spores incubated with taurocholate ( Fig. 4a ). Interestingly, although high concentrations of deoxycholate (1.0%) can trigger germination of C. difficile spores [20] , at the concentrations tested here germination levels were significantly lower than what was observed in response to taurocholate ( Fig. 4a ). 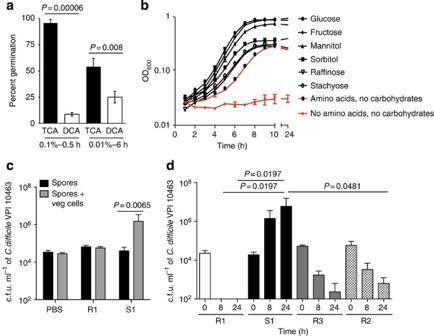Figure 4:C. difficile in vitroandex vivogermination and growth studies. (a)In vitroassays to assess the ability of taurocholate (black bars) and deoxycholate (white bars) to triggerC. difficilespore germination. Spores were incubated in BHIS with each bile salt at the indicated concentrations. Spores were incubated with 0.1% bile salt for 30 min or with 0.01% bile salt for 6 h. Data presented represent mean±s.d. of triplicate experiments and were significant (Student’st-test). (b)In vitrogrowth ofC. difficilein a defined minimal media, which included essential amino acids and vitamins required byC. difficilefor growth. Carbohydrates that were found to be increased after antibiotic treatment during the CDI-susceptible state (S1) were supplemented in the media.C. difficilecan utilize many of the carbohydrates in the murine gut after antibiotic treatment. Only carbohydrates that supported growth ofC. difficileare shown here (Supplementary Table 1). Error bars represent the mean±s.e.m. of triplicate experiments. (c)Ex vivogermination and outgrowth ofC. difficilein caecal contents from untreated and from cefoperazone-treated mice 2 days after antibiotics.C. difficileVPI 10463 spores inoculated into the antibiotic-treated caecal contents (S1,n=6) were able to germinate and outgrow over a 6-h period, whereas spores in the non-antibiotic-treated caecal content (R1,n=3) did not. Significance between groups was done by the Mann–Whitney non-parametrict-test. Error bars represent the mean±s.e.m. (d)Ex vivogrowth ofC. difficileVPI 10463 in mouse caecal content from all four treatment groups representing all environmental states (R1, S1, R3 and R2).C. difficilevegetative cells were able to grow to high levels over a 24-h period in the contents from mice in the susceptible state (S1) compared with contents from mice in the resistant states (R1, R2 and R3). Data presented represent mean±s.d. of triplicate experiments and were significant by non-parametric Kruskal–Wallis one-way analysis of variance test followed by the Bonferroni–Dunn multiple comparison test. Figure 4: C. difficile in vitro and ex vivo germination and growth studies. ( a ) In vitro assays to assess the ability of taurocholate (black bars) and deoxycholate (white bars) to trigger C. difficile spore germination. Spores were incubated in BHIS with each bile salt at the indicated concentrations. Spores were incubated with 0.1% bile salt for 30 min or with 0.01% bile salt for 6 h. Data presented represent mean±s.d. of triplicate experiments and were significant (Student’s t -test). ( b ) In vitro growth of C. difficile in a defined minimal media, which included essential amino acids and vitamins required by C. difficile for growth. Carbohydrates that were found to be increased after antibiotic treatment during the CDI-susceptible state (S1) were supplemented in the media. C. difficile can utilize many of the carbohydrates in the murine gut after antibiotic treatment. Only carbohydrates that supported growth of C. difficile are shown here ( Supplementary Table 1 ). Error bars represent the mean±s.e.m. of triplicate experiments. ( c ) Ex vivo germination and outgrowth of C. difficile in caecal contents from untreated and from cefoperazone-treated mice 2 days after antibiotics. C. difficile VPI 10463 spores inoculated into the antibiotic-treated caecal contents (S1, n =6) were able to germinate and outgrow over a 6-h period, whereas spores in the non-antibiotic-treated caecal content (R1, n =3) did not. Significance between groups was done by the Mann–Whitney non-parametric t -test. Error bars represent the mean±s.e.m. ( d ) Ex vivo growth of C. difficile VPI 10463 in mouse caecal content from all four treatment groups representing all environmental states (R1, S1, R3 and R2). C. difficile vegetative cells were able to grow to high levels over a 24-h period in the contents from mice in the susceptible state (S1) compared with contents from mice in the resistant states (R1, R2 and R3). Data presented represent mean±s.d. of triplicate experiments and were significant by non-parametric Kruskal–Wallis one-way analysis of variance test followed by the Bonferroni–Dunn multiple comparison test. Full size image To examine the ability of various nutrients to support the growth of C. difficile , we carried out in vitro growth studies using a defined minimal media, which included essential amino acids and vitamins. Our metabolomic data indicated that levels of sorbitol, mannitol, arabitol, xylitol, gluconate, sucrose, lactate, raffinose, stachyose, galactose and fructose were increased in the state susceptible to CDI ( Figs 2c and 3b ). Therefore, we tested the ability of C. difficile to utilize each of these sugars, compared with growth on glucose. In media supplemented with glucose, fructose, mannitol or sorbitol, C. difficile exhibited decreased growth lag, increase in growth rate and a higher final cell density compared with the controls without additional carbohydrate ( Fig. 4b ). In contrast, C. difficile grown in raffinose and stachyose exhibited decreased growth lag but failed to increase maximal growth rate and final density compared with the no carbohydrate control ( Fig. 4b ). All other carbohydrates tested had negligible effects of the growth dynamics compared with growth on amino acids without a carbohydrate source ( Supplementary Table 1 ). These results demonstrate that C. difficile can utilize the specific metabolites detected in the targeted metabolomics approach for germination and growth and at the same physiological concentrations. To determine whether similar effects could be observed in the complex environment encountered in the murine gut, we harvested the caecal contents from mice with and without antibiotic treatment. The caecal contents from these mice were tested to determine whether they would support germination and outgrowth of C. difficile spores and growth of vegetative C. difficile ex vivo . Within 6 h, spores of C. difficile strain VPI 10463 were able to germinate and initiate outgrowth in the caecal content of mice treated with antibiotics compared with non-antibiotic control mouse caeca ( Fig. 4c ). To directly test the ability of vegetative C. difficile cells to grow in the caecal content of mice following antibiotics, we monitored growth of C. difficile VPI 10463 over a 24-h period (at time 0, 8 and 24 h) in caecal contents from mice in each of the functional states depicted in Fig. 1 . Only caecal content from mice in state S1 (2 days after cefoperazone treatment, which corresponded to clinical loss of colonization resistance) supported growth of vegetative C. difficile 24 h after inoculation ( Fig. 4d ). Vegetative cells inoculated into the caecal contents from mice with the resistant states did not exhibit growth. In fact, the number of colony-forming units decreased over 24 h suggesting a loss of viability of the inoculum. These were not strain-dependent effects as similar results were seen with spores and vegetative cells of the current epidemic strain of C. difficile (BI/NAP1/027) ( Supplementary Fig. 7 ). Correlations between the gut microbiome and metabolome The concomitant alterations of the microbiome (84 operational taxonomic units (OTUs)) and metabolome composition (480 metabolites) across the four experimental groups suggested the presence of widespread associations between the two data types. To examine such associations, we calculated the Spearman’s rank correlation coefficient ρ (‘rho’) for all OTU-metabolite pairs ( Fig. 5a ) using the data across the same 30 samples. To visualize these correlations, we first performed unsupervised clustering of OTUs, which revealed four clusters (O1–O4, Supplementary Data 3 ), which were used to order these OTUs in the sample-OTU matrix ( Fig. 5c ). Similarly, unsupervised clustering of metabolites uncovered two major clusters (M1–M2, Supplementary Data 4 ). Within each cluster, we grouped metabolites according to their pathway annotations and used this metabolite order to organize the sample-metabolite matrix ( Fig. 5b ). Examination of the correlations organized in this manner revealed distinctive relationships between OTUs and metabolites in the different environmental states. For example, OTUs in the first OTU cluster (O1) were positively correlated with the metabolites in the first metabolite cluster (M1) as both O1 and M1 had low values in R1 and R2 samples, increased in the susceptible state S1 samples and returned to low values in R3 samples. Metabolites present in metabolite cluster M1 and OTU cluster O1 included taurocholate, carbohydrates and amino acids, all metabolites that C. difficile could utilize for germination and growth in vitro ( Fig. 4a,b , Supplementary Data 4 ). This is in contrast to the negative correlation between O1 and M2, which were reduced in the S1 state. Two other OTU clusters, O2 and O4, were similar in that they both contained OTUs that were reduced in S1 and negatively correlated with M1 metabolites. The last cluster, O3, was similar to O2 and O4 in having OTUs that were reduced in S1. However, unlike O2/O4, O3 OTUs contained predominantly members of the Bacteroidetes phylum, and were not recovered in the resistant state R3. 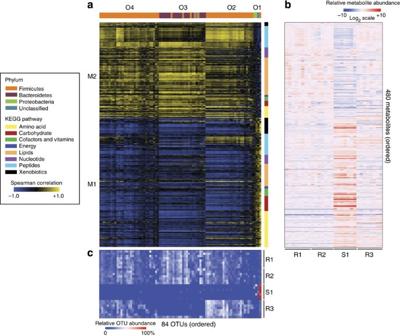Figure 5: Correlation analysis of the microbiome and metabolome. (a) Spearman’s correlation analysis was done with all 84 OTUs in the microbiome colour coded by phylum and grouped based on unsupervised clustering. All 480 metabolites in the metabolome were similarly clustered and then colour coded by KEGG super pathway. There were four distinct clusters of OTUs that were seen, O1–O4, and two distinct clusters of metabolites, M1–M2. The heatmap scale ranges from +1.0 to −1.0. (b) Relative levels of metabolites from all treatment groups (R1, R2, S1 and R3) depicted in a heatmap but keeping with the same order of metabolites as ina. The heatmap scale for relative levels of metabolites ranges from +10 to −10 on a log2scale. (c) Relative abundance of OTUs from all treatment groups (R1, R2, S1 and R3) is depicted in a heatmap but keeping with the same order of OTUs as ina. The heatmap scale ranges from 0–100% relative abundance. Figure 5: Correlation analysis of the microbiome and metabolome. ( a ) Spearman’s correlation analysis was done with all 84 OTUs in the microbiome colour coded by phylum and grouped based on unsupervised clustering. All 480 metabolites in the metabolome were similarly clustered and then colour coded by KEGG super pathway. There were four distinct clusters of OTUs that were seen, O1–O4, and two distinct clusters of metabolites, M1–M2. The heatmap scale ranges from +1.0 to −1.0. ( b ) Relative levels of metabolites from all treatment groups (R1, R2, S1 and R3) depicted in a heatmap but keeping with the same order of metabolites as in a . The heatmap scale for relative levels of metabolites ranges from +10 to −10 on a log 2 scale. ( c ) Relative abundance of OTUs from all treatment groups (R1, R2, S1 and R3) is depicted in a heatmap but keeping with the same order of OTUs as in a . The heatmap scale ranges from 0–100% relative abundance. Full size image The concerted changes within the microbiome and metabolome allowed us to construct interaction networks for both OTUs and metabolites using the strongest pairwise correlations (see Methods). The resulting networks were functionally coherent. In the microbiome, there were two OTU subnetworks that were connected with each other within the microbiome ( Supplementary Fig. 8a ), one consisting of members from both the Bacteroidetes and Firmicutes phyla and another that was solely made up of members of the Firmicutes phyla. In the metabolome ( Supplementary Fig. 8b ), there were four metabolite subnetworks that were connected with each other and were functionally distinct in that three were enriched for lipids, peptides and amino acids, respectively, and the fourth contained a mixture of carbohydrates, xenobiotics and peptides. Juxtaposition of the inferred networks for OTUs ( Supplementary Fig. 8a ) and metabolites ( Supplementary Fig. 8b ) revealed strong connections between the gastrointestinal microbiota and the metabolome. Both networks from the microbiome, Bacteroidetes/Firmicutes and Firmicutes, were positively correlated with lipids and peptides and negatively correlated with amino acids and the carbohydrate/xenobiotic/peptide group. An OTU, not shown in Supplementary Fig. 8 , is from the Firmicutes phylum and Lactobacillaceae family and was most abundant during the susceptible state of CDI (S1; see cluster O1 in Fig. 5a ). It had the exact opposite correlations with metabolites and OTUs (lipids ρ =−0.40, peptides ρ =−0.33; amino acids ρ =0.73; carbohydrates/xenobiotics/peptides ρ =0.73). These results indicate that the metabolites in the gut, especially ones that C. difficile can utilize for germination and growth, were strongly affected by members of the two dominant phyla, Firmicutes and Bacteroidetes. Two completely different microbial communities dominated by different phyla can have similar metabolic relationships and similar outcomes of disease. To link microbiome community structure to function in the setting of CDI, we undertook a multi-omics approach to characterize the changes in the murine gut microbiome and metabolome following antibiotic administration. By determining whether the intestinal ecosystem would support the colonization of C. difficile , we determined that at least two distinct community structures had complete colonization resistance against the pathogen. Although these two resistant community structures had observable differences with regard to the total metabolome, they were indistinguishable with respect to primary and secondary bile acids, carbohydrates and fatty acids. We integrated analysis of the microbiome structure and function with measurements of pertinent aspects of C. difficile physiology (focusing on germination and vegetative growth) to obtain a more global view of the dynamics of the intestinal ecosystem in the setting of CDI. This study is the first to identify specific metabolites that are present in situ within the altered gut environment that C. difficile can utilize for germination and growth and thus could act as a key mechanistic link between antibiotic use and C. difficile susceptibility. In addition, our ex vivo results suggest that the normal gut environment can be directly inhibitory to the pathogen. One candidate for such an inhibitory metabolite would be the secondary bile acid deoxycholate. This metabolite is elevated in the baseline metabolome and has been shown to be inhibitory to vegetative C. difficile [20] . Previous studies have indicated that antibiotic treatment can alter the relative abundance of bile acids within the intestinal environment [26] , [27] . Our results indicate that bile acids may play key roles in modulating the pathogenesis of C. difficile in vivo , affecting multiple aspects of pathogen physiology. This study also indicates that multiple community structures of the microbiome can share a similar function [28] , as suggested that individuals may possess one of several enterotypes distinguished by dominant microbiome members [29] , but all have normal gastrointestinal health. Implied in this concept is the fact that bacteria can share specific functions such as the ability to deconjugate primary bile acids or ferment carbohydrates into SCFAs across the taxonomic spectrum. We determined that the ability to metabolize bile acids and ferment carbohydrates into SCFAs could be carried out both by a community with an equal abundance of Firmicutes and Bacteroidetes as well as one that is dominated by Firmicutes alone ( Fig. 5 ). These results underscore the importance of looking beyond microbiome community structure and measuring functional aspects when determining the relationship between the microbiome and human health and disease. Our ability to gain insight into the metabolic function of the microbiome, using metabolomic approaches as we have done in this study, or metagenomic [30] , [31] or metaproteomic [32] , characterization should lead to diagnostic and therapeutic modalities targeting the microbiome in response to CDI and other diseases. Animals and housing C57BL/6 WT mice (5- to 14-week old; male or female) were used from a breeding colony that was established using animals purchased from Jackson Laboratories for the experimental infections. Mice were housed with autoclaved food, bedding and water. Cage changes were performed in a laminar flow hood. Mice had a cycle of 12 h of light and 12 h of darkness. The University Committee on the Care and Use of Animals at the University of Michigan approved this study. The University of Michigan laboratory animal care policies follow the Public Health Service policy on Humane Care and Use of Laboratory Animals. Animals were assessed twice daily for physical condition and behaviour and those assessed as moribund were humanely euthanized by CO 2 asphyxiation. Trained animal technicians performed animal husbandry in an AAALAC-accredited facility. C. difficile spore preparation C. difficile VPI 10463 (ATCC 43255) spores were prepared as follows. C. difficile VPI 10463 was grown overnight in a 2-ml culture of Columbia Broth at 37 °C anaerobically. The next day, the inoculum was added to 40 ml culture of Clospore media [33] . The culture was incubated at 37 °C for 5–7 days anaerobically. Spores were harvested by centrifugation and washed with cold water at least three times. Spore stocks were stored at 4 °C in sterile water. C. difficile spores were heat treated for 20 min at 65 °C to ensure that any remaining vegetative bacilli were killed before gavaging animals. Viable spores were enumerated by plating for colony-forming units (c.f.u.) ml −1 on taurocholate, cefoxitin, cycloserine, fructose agar (TCCFA) to determine the challenge dose. Antibiotic administration and challenge with C. difficile C57BL/6 WT mice (male or female) ranging from 5–14 weeks in age were used in this study. Two groups of mice ( n =20 per group) were given cefoperazone (0.5 mg ml −1 ) in sterile drinking water for 10 days and allowed either 2 days (S1) or 6 weeks of recovery (R3) on regular drinking water. Two other groups of mice ( n =20 per group) were given sterile drinking water during the duration of these experiments as non-antibiotic controls (R1 and R2). Mice ( n =8) from each treatment were euthanized by CO 2 asphyxiation and necropsied the same day that cohoused mice from the same treatment groups were challenged with 250 C. difficile VPI 10463 spores by oral gavage. Caecal content and tissue snips were collected at the time of necropsy and flash frozen for microbiome and metabolome analysis. Cohoused animals challenged with C. difficile were monitored for signs of clinically severe CDI including inappetence, diarrhoea and hunching. Animals were euthanized by CO 2 asphyxiation after losing 20% of initial baseline weight or after developing all severe clinical signs listed above. At the time of necropsy (2 days post infection), bacterial enumeration was done from the caecal content of animals infected with C. difficile on TCCFA selective agar to quantitate levels of colonization. Microbiome analysis DNA extraction was done on murine caecal tissue snips that included luminal content using Roche MagNA Pure Compact system. Sample processing was done according to the Roche MagNA Pure Nucleic Acid Isolation Kit I protocol instructions. Fold change of total 16S rRNA genes as a proxy for bacterial load in untreated and cefoperazone-treated mice was done by quantitative PCR [6] . Values represent relative abundance of the bacterial 16S rRNA-coding region normalized to host DNA content, using a single-copy mouse gene (encoding, tumour necrosis factor (TNF)α). In brief, quantitative PCR assays used the LightCycler 480 Probes Master reaction mixture (Roche) at 1 × concentration with appropriate primer-probe sets (100 nmol for each primer and probe) and sample DNA (100 ng). Sequences for the forward primer (5′-TCCTACGGGAGGCAGCAGT-3′), the reverse primer (5′-GGACTACCAGGGTATCTAATCCTGTT-3′) and the probe (5′-[6-carboxyfluorescein]-CGTATTACCGCGGCTGCTGGCAC-[6-carboxytetramethylrhodamine]-3′) were based on the work of Nadkarni et al. [34] Final assay volumes of 20 μl were dispensed in triplicate into 96-well plates and repeated in duplicate. Signals were detected with a LightCycler 480 instrument (Roche). The reaction conditions for the amplification of DNA were 95 °C for 10 min and 40 cycles of 95 °C for 15 s and 60 °C for 1 min. Detection of the host signal used 200 nmol of the forward (TNFa_mu_se; 5′-GGCTTTCCGAATTCACTGGAG-3′) and reverse (TNFa_mu_as; 5′-CCCCGGCCTTCCAAATAAA-3′) primers and 100 nmol of the probe (TNFa_mu_probe; 5′-Cy5-ATGTCCATTCCTGAGTTCTGCAAAGGGA-Iowa Black RQ-3′), adapted from the work of Nitsche et al. [35] Amplification of the host signal began with incubation at 95 °C for 10 min, followed by 45 cycles of 95 °C for 20 s and 64 °C for 30 s. Relative bacterial loads were compared via the ΔΔ C T method by normalizing the 16S signal to the host signal. Amplification of the V3–V5 region of the 16S rRNA gene was accomplished using the Broad HMP protocol (HMP MDG Default Protocol v4.2), which can be found at http://www.hmpdacc.org/doc/16S_Sequencing_SOP_4.2.2.pdf . In brief, extracted DNA was used to construct DNA libraries targeting the V3–V5 hypervariable regions of the 16S rRNA gene using primers 357F (5′-CCTACGGGAGGCAGCAG-3′) with a B adaptor (5′-CCTATCCCCTGTGTGCCTTGGCAGTCTCAG-3′) and 926R (5′-CCGTCAATTCMTTTRAGT-3′) with a unique barcode to identify the target and an A adaptor (5′-CCATCTCATCCCTGCGTGTCTCCGACTCAG-3′). A PCR reaction mixture of 1X AccuPrime PCR Buffer II (Invitrogen), 0.15 μl AccuPrime Taq DNA Polymerase High Fidelity, 0.2 μM primer B, 0.2 μM uniquely barcoded Primer A was used. DNA was amplified using the following conditions: 95 °C for 2 min, 30 cycles of 95 °C for 20 s, 50 °C for 30 s and 72 °C for 5 min. Amplicons were cleaned with the Agencourt AMPure XP (Beckman Coulter Inc.) and quantified using the Quant-it PicoGreen dsDNA kit (Invitrogen). Samples were pooled in equal proportion, cleaned again with AMPureXP (Agilent) and sequenced on the Roche 454 GS Junior Titanium platform according to the manufacturer’s specifications. Analysis of 454-pyrosequencing data was done using mothur (version 1.25.1) [36] . In brief, instructions from SOP (standard operating procedure) at the website http://www.mothur.org/wiki/Schloss_SOP were followed to process pyrosequencing data. We used mothur to group or assign 16S rRNA bacterial sequences into OTUs using a 3% species level definition. Classifications were determined by comparing sequences to the Ribosomal Database Project [37] . Classified OTUs were used to determine the relative abundance of bacterial phyla and family in each sample. Principal coordinates analysis was used to assess community similarity among all samples and was calculated [38] . This ordination was generated using a Yue and Clayton-based distance matrix representing the relative abundance of OTUs in each community at a 3% OTU definition level. The distances between the communities were displayed in a two-dimensional space. Analysis of the V3–V5 region of the 16S rRNA gene yielded a total of 94,708 raw sequence reads. The sequence data have been deposited in the SRA database under the SRA study SRP033403. Following trimming and chimera removal, a total of 41,368 sequences with minimum read length at 245 base pairs were used in the final analysis. From these sequences, we detected a total of 791 OTUs with a definition of >97% sequence similarity. To focus on the most abundant OTUs (which should be the most important from a metabolic standpoint based on mass action), the OTU data were then filtered to include only those OTUs that made up 1% or more of the total sequences. After filtering the final number of OTUs was 84. Heatmaps of microbiome data (OTUs) were made using the heatmap command in R (ref. 39 ). The heatmap command reorders the data in the rows, and the columns separately, so that similar data are grouped together by hierarchical clustering, as shown by dendrograms for the rows and the columns. The Euclidean distance was used in the clustering [40] . Untargeted metabolomic analysis Metabolomic profiling analysis was performed by Metabolon (Durham, NC) [23] in the following way. Each sample was accessioned into the Metabolon laboratory information management system (LIMS) system and was assigned by the LIMS a unique identifier that was associated with the original source identifier only. This identifier was used to track all sample handling, tasks, results and so on. The samples (and all derived aliquots) were tracked by the LIMS system. All portions of any sample are automatically assigned their own unique identifiers by the LIMS when a new task is created; the relationship of these samples is also tracked. All samples were maintained at −80 °C until processed. Samples were prepared using the automated MicroLab STAR system from Hamilton Company. A recovery standard was added before the first step in the extraction process for quality control (QC) purposes. Sample preparation was conducted using aqueous methanol extraction process to remove the protein fraction while allowing maximum recovery of small molecules. The resulting extract was divided into four fractions: one for analysis by ultrahigh performance liquid chromatography/mass spectroscopy (UPLC/MS/MS; positive mode), one for UPLC/MS/MS (negative mode), one for GC/MS and one for backup. Samples were placed briefly on a TurboVap (Zymark) to remove the organic solvent. Each sample was then frozen and dried under vacuum. Samples were then prepared for the appropriate instrument, either UPLC/MS/MS or GC/MS. The LC/MS portion of the platform was based on a Waters ACQUITY ultra-performance liquid chromatography (UPLC) and a Thermo-Finnigan linear trap quadrupole mass spectrometer, which consisted of an electrospray ionization source and linear ion-trap mass analyser [41] . The sample extract was dried and then reconstituted in acidic or basic LC-compatible solvents, each of which contained eight or more injection standards at fixed concentrations to ensure injection and chromatographic consistency. One aliquot was analysed using acidic positive ion-optimized conditions and the other using basic negative ion-optimized conditions in two independent injections using separate dedicated columns. Extracts reconstituted in acidic conditions were gradient eluted using water and methanol containing 0.1% formic acid, while the basic extracts, which also used water/methanol, contained 6.5 mM ammonium bicarbonate. The MS analysis alternated between MS and data-dependent MS [2] scans using dynamic exclusion. Raw data files were archived and extracted as described below. The samples destined for GC/MS analysis were re-dried under vacuum desiccation for a minimum of 24 h before being derivatized under dried nitrogen using bistrimethyl-silyl-triflouroacetamide. The GC column was 5% phenyl and the temperature ramp was from 40° to 300 °C in a 16-min period. Samples were analysed on a Thermo-Finnigan Trace DSQ fast-scanning single-quadrupole mass spectrometer using electron impact ionization. The instrument was tuned and calibrated for mass resolution and mass accuracy on a daily basis. The information output from the raw data files was automatically extracted as discussed below. For quality assurance/QC purposes, additional samples were included with each day’s analysis. These samples included extracts of a pool of well-characterized human plasma, extracts of a pool created from a small aliquot of the experimental samples and process blanks. QC samples were spaced evenly among the injections and all experimental samples were randomly distributed throughout the run. A selection of QC compounds was added to every sample for chromatographic alignment, including those under test. These compounds were carefully chosen so as not to interfere with the measurement of the endogenous compounds. Raw data were extracted, peak identified and QC processed using Metabolon’s hardware and software. These systems are built on a web service platform utilizing Microsoft’s .NET technologies, which run on high-performance application servers and fibre-channel storage arrays in clusters to provide active failover and load balancing [42] . Compounds were identified by comparison with library entries of purified standards or recurrent unknown entities. More than 2,400 commercially available purified standard compounds have been acquired and registered into LIMS for distribution to both LC and GC platforms for determination of their analytical characteristics. In all, a data set of 480 annotated compounds was delivered. Pathways were assigned for each metabolite, allowing examination of overrepresented pathways. For statistical analysis, missing values (if any) are assumed to be below the level of detection. However, biochemicals that were detected in all samples from one or more groups but not in samples from other groups were assumed to be near the lower limit of detection in the groups in which they were not detected. In this case, the lowest detected level of these biochemicals was imputed for samples in which that biochemical was not detected. Following log transformation and imputation with minimum observed values for each compound, we further normalized the entire set of 32 samples so that the median value of absolute mass across 480 annotated metabolites was centred across samples. Welch’s two-sample t -test was used to identify biochemicals that differed significantly between experimental groups. We defined significantly different compounds between treatment groups by the criteria of fold change>2 × and P -value<0.05. To display the between-group comparison results of all metabolites, we generated ‘volcano plots’ in R, with fold change on the x axis and −log( P -value) on the y axis. Metabolites that increased by twofold or more and had a P <0.05 were shown in red, whereas those decreased by twofold or more and had a P <0.05 were shown in green ( Supplementary Fig. 6 ). Targeted metabolomic analysis For targeted metabolomic data, caecal content from mice was weighed at necropsy and flash frozen in liquid nitrogen. Samples were sent to the Michigan Regional Comprehensive Metabolomics Resource Core. Caecal samples were dispersed in acidified water spiked with stable isotope-labelled SCFA standards, and then extracted with diethyl ether. The ether layer was immediately analysed by gas chromatography/mass spectroscopy using a Phenomenex ZB-WAX column on an Agilent 6890 GC with a 5973MS detector. Quantitation was performed by calibration to internal standards. The bile acids were detected by negative LC-electrospray ionization-triple quadrupole (QqQ) mass spectrometry and three of them (lithocholic acid, chenodeoxycholic acid and ursodeoxycholic acid) were detected by positive mode. Quantitation was performed by calibration to internal standards. Extraction of carbohydrates (mannitol and sorbitol) was done using a combination of a modified Bligh–Dyer procedure to remove lipids followed by protein precipitation by adding methanol to aqueous phases [43] . LC-MS instruments used in this work included the Agilent 1200 HPLC, a quadrupole time of flight MS/MS (6530) and a QqQ MS/MS (6450) system. Both quadrupole time of flight and QqQ instruments were optimized for the highest mass accuracy and sensitivity for carbohydrate detection in the negative mode. Data acquisition and data processing was done using the Agilent Technologies MassHunter Workstation and Quantitative Analysis Software. Microbiome and metabolome correlation analysis We computed the Spearman rank correlation coefficients ( ρ ) for all pairs among the 480 metabolites and focused on strong positive interactions with ρ >0.9. This resulted in a sparse matrix of 800 interactions involving 157 unique metabolites. We performed network analysis of the interaction matrix using the fastgreedy.community algorithm in the R package igraph [39] . This algorithm identifies subgraphs using direct optimization of a modularity score. Each discovered community was annotated according to the KEGG pathways of the metabolites within the community. In parallel, we calculated ρ for the 84 OTUs. Applying a filter of 0.7 resulted in 307 interactions among 63 unique OTUs in the interaction matrix. To examine the interaction between metabolites and OTUs, we also computed the ρ matrix between the 157 metabolites and the 63 OTUs ( Supplementary Fig. 8 ). We similarly performed network construction in igraph and annotated each community by the phylum that the OTUs belong to. C. difficile in vitro germination assays To assess germination of C. difficile spores in response to specific compounds, we took advantage of the fact that C. difficile spores are unable to germinate in the absence of taurocholate on brain heart infusion (BHIS) plus 100 mg l −1 L -cysteine agar alone. Spores were subjected to heat treatment (65 °C for 20 min) before use for these studies. Germination was assayed by comparing growth on BHIS plates (vegetative cells only) with growth on BHIS agar supplemented with 0.1% taurocholate (total c.f.u.). Purified VPI 10463 spores were incubated in BHIS supplemented with either taurocholate or deoxycholate at specified concentration for indicated times before dilution plating for c.f.u. Percent germination was calculated as [(c.f.u. on BHIS)/(c.f.u. on BHIS+taurocholate) × 100]. Germination under each condition was performed in triplicate. C. difficile in vitro growth curves with carbohydrates No carbon minimal medium (NCMM) is modified from the basal defined medium [24] . To examine the growth of C. difficile from various carbohydrates, the modification of basal defined medium was necessary to decrease the utilization of amino acids as carbon sources. NCMM utilizes the vitamins and amino acids at the following concentrations: biotin, 0.125 mg l −1 ; pyridoxine and pantothenate, 1 mg l −1 ; histidine, glycine and tryptophan, 75 mg l −1 ; arginine, methionine and threonine 150 mg l −1 ; valine and isoleucine, 225 mg l −1 ; leucine, 300 mg l −1 ; cysteine, 400 mg l −1 ; and proline, 450 mg l −1 . Various carbohydrates were added individually at a concentration of 5,000 mg l −1 . C. difficile VPI 10463 was cultured overnight at 37 °C in BHIS plus 100 mg l −1 L -cysteine in an anaerobic growth chamber (Coy Labs). After 14 h of growth, C. difficile was subcultured 1:3 into NCMM+0.5% glucose and allowed to grow for 3 h anaerobically at 37 °C. The culture was centrifuged anaerobically at 2,000 × g for 10 min and resuspended in an equal volume of anaerobically equilibrated 1 × PBS buffer. An aliquot of 100 μl of this suspension was used to inoculate 5 ml of NCMM with 0.5% of the appropriate carbohydrate. Medium was placed in anaerobic vials and sealed with gas impermeable, butyl rubber stoppers [44] . Tubes were removed from the anaerobic chamber and incubated at 37 °C with shaking at 200 r.p.m. Cell density (OD 600 ) was monitored hourly in a Thermo Scientific Spectronic 20D+ apparatus. The specific growth rate was determined as μ =ln( X/X o )/ T , where X is the OD 600 value during the linear portion of growth and T is time in hours. Values given are the mean μ values of three independent cultures done twice ( Supplementary Table 1 ). Ex vivo germination and growth studies in mouse caecal contents Spores were subjected to heat treatment (65 °C for 20 min) before use for these studies. Mouse caecal content (non-antibiotic and antibiotic treated) was weighed passed into an anaerobic chamber and diluted 1:1 ratio with PBS. C. difficile spores were added to PBS-diluted murine caecal content and a PBS-only control, and then incubated at 37 °C anaerobically for 6 h to assess germination and outgrowth. After incubation, bacterial enumeration was done on TCCFA selective media. The remaining caecal content was heated at 65 °C for 20 min to kill off any vegetative cells and then bacterial enumeration was done. Samples plated without heating represent spores and vegetative cells (germination and outgrowth). Samples plated with heat treatment represent spore counts only. Ex vivo growth studies were done in a similar manner. Mouse caecal content from various treatments (R1–R3 and S1) was prepared and diluted with PBS as described above. Caecal content was inoculated with ~10 4 c.f.u. of C. difficile vegetative cells and incubated at 37 °C anaerobically for 24 h. In brief, an overnight culture of C. difficile was diluted 1:10 and then allowed to grow for 2 h at which point cells were properly diluted again and added to caecal content. Samples were taken at time points 0, 8, and 24 h and bacterial enumeration was done on TCCFA plates to define growth over a 24-h period. Accession codes: The sequence data have been deposited in the SRA database under accession code SRP033403 . How to cite this article: Theriot, C. M. et al. Antibiotic-induced shifts in the mouse gut microbiome and metabolome increase susceptibility to Clostridium difficile infection. Nat. Commun. 5:3114 doi: 10.1038/ncomms4114 (2014).